Visible-light photoredox-catalyzed umpolung carboxylation of carbonyl compounds with CO2 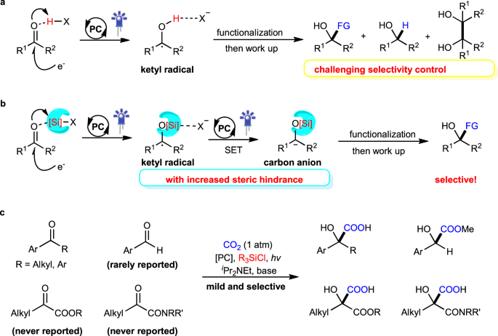Fig. 1: Strategies for umpolung functionalization of carbonyl compounds via photocatalysis. aPrevious strategy: proton-coupled electron transfer via photocatalysis.bOur design: chlorosilane-coupled electron transfer via photocatalysis.cThis work: a general umpolung carboxylation of carbonyls via photocatalysis. FG functional groups, PC photocatalyst. Photoredox-mediated umpolung strategy provides an alternative pattern for functionalization of carbonyl compounds. However, general approaches towards carboxylation of carbonyl compounds with CO 2 remain scarce. Herein, we report a strategy for visible-light photoredox-catalyzed umpolung carboxylation of diverse carbonyl compounds with CO 2 by using Lewis acidic chlorosilanes as activating/protecting groups. This strategy is general and practical to generate valuable α-hydroxycarboxylic acids. It works well for challenging alkyl aryl ketones and aryl aldehydes, as well as for α-ketoamides and α-ketoesters, the latter two of which have never been successfully applied in umpolung carboxylations with CO 2 (to the best of our knowledge). This reaction features high selectivity, broad substrate scope, good functional group tolerance, mild reaction conditions and facile derivations of products to bioactive compounds, including oxypheonium, mepenzolate bromide, benactyzine, and tiotropium. 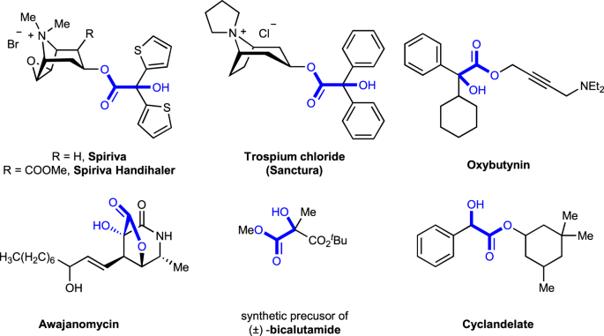Fig. 2: The significance of α-Hydroxycarboxylic acids. Selected examples of bioactive molecules and natural products that containing α-Hydroxycarboxylic acids moiety. Moreover, the formation of carbon radicals and carbanions as well as the key role of chlorosilanes are supported by control experiments. Carbonyl compounds, especially ketones and aldehydes, are important bulk chemicals in industry and they exist widely in natural products, pharmaceuticals, and materials. The electronic structure of the carbonyl group renders it sensitive to attack from nucleophiles at the carbon center. Different from the inherent reactivity, the umpolung strategy has been investigated extensively to achieve C–C and C–X bond formations with non-nucleophilic reaction partners [1] , [2] , [3] . Notably, significant attention has been paid to recent progress in visible-light-driven umpolung reactions of carbonyl compounds owing to their mild reaction conditions and green processes [2] , [3] . In addition to direct single electron transfer (SET) reduction of carbonyls [4] , the photocatalytic proton-coupled electron transfer (PCET) [5] approach represents a powerful tool for SET reduction of unactivated carbonyls to generate ketyl radicals (Fig. 1a ), which then could undergo diverse transformations, including ketyl-olefin/alkyne coupling [6] , [7] , [8] , [9] , [10] , ketyl-ketyl homocoupling (pinacol coupling) [11] , and other couplings [12] , [13] , [14] , [15] , [16] . Such electron-rich ketyl radical intermediates, however, rarely undergo a second photocatalytic SET reduction process to produce a carbanionic species [17] , [18] , [19] , [20] . Meanwhile, the introduction of protons can accelerate pinacol coupling side reactions [20] . We envisioned the photoredox-catalyzed umpolung functionalization of carbonyl groups by using the Lewis acidic chlorosilane as an activating/protecting groups (Fig. 1b ). Fig. 1: Strategies for umpolung functionalization of carbonyl compounds via photocatalysis. a Previous strategy: proton-coupled electron transfer via photocatalysis. b Our design: chlorosilane-coupled electron transfer via photocatalysis. c This work: a general umpolung carboxylation of carbonyls via photocatalysis. FG functional groups, PC photocatalyst. Full size image α-Hydroxycarboxylic acids are highly important motifs in pharmaceutical and polymer industries (Fig. 2 ) [21] , [22] , [23] , [24] , [25] , [26] , [27] , [28] , [29] . As traditional methods through cyanation and hydrolysis suffer from the use of toxic cyanide and harsh conditions, chemists have long searched for more sustainable synthetic routes [30] . Compared to cyanide and carbon monoxide, CO 2 represents a better choice as a C1 source in carboxylation due to its abundance, nontoxicity, and recyclability [31] , [32] , [33] , [34] , [35] , [36] , [37] , [38] , [39] . Although significant progress has been achieved in recent decades to generate α-hydroxycarboxylic acids with CO 2 [18] , [19] , [20] , [40] , [41] , [42] , [43] , most of these methods suffer from the utilization of stoichiometric amounts of metal reductants, low functional group tolerance, limited substrate scope, and/or competitive side reactions, especially the pinacol coupling and reduction, thus hampering industrial application. Therefore, a general and practical method is desirable. Inspired by recent visible-light-driven reductive carboxylations of different electrophiles with CO 2 [44] , [45] , [46] , [47] , [48] , [49] , [50] , [51] , [52] , [53] , [54] , [55] , [56] , [57] , [58] , [59] , we wondered whether we could develop a general and practical strategy to achieve efficient and selective carboxylation of carbonyls with CO 2 via visible-light photoredox catalysis. Achieving such a goal requires addressing several challenges. First, it is highly challenging to avoid common side reactions, namely pinacol coupling [11] and hydrogen atom transfer (HAT) of ketyl radicals [60] . Second, as the direct radical addition of ketyl radicals to CO 2 is less favored [61] , [62] , a second SET reduction to generate a carbanion, which could attack electrophilic CO 2 , would be promising. However, the direct SET reduction of electron-rich ketyl radicals and/or ketyl radical anions is challenging. Third, it is very difficult to avoid other processes, including direct α-carboxylation [63] and homo-aldol reaction [64] of alkyl ketones, as well as the disproportionation [65] of aldehydes (Cannizzaro reaction) under basic conditions. Here, we show a general and practical reductive carboxylation of carbonyl compounds, such as alkyl aryl ketones, diaryl ketones, α-ketoamides, α-ketoesters, and aryl aldehydes, with CO 2 to give valuable α-hydroxycarboxylic acids (Fig. 1c ). Fig. 2: The significance of α-Hydroxycarboxylic acids. Selected examples of bioactive molecules and natural products that containing α-Hydroxycarboxylic acids moiety. Full size image With such challenges in mind, we were inspired by PCET [5] and hypothesized whether we could use a Lewis acidic chlorosilane instead of a proton as an activating group to promote the visible light-driven SET reduction of a carbonyl group, which has never been reported yet. Moreover, the activating chlorosilane might act as a temporary protecting group to generate α-silyloxy carbon radicals, which would increase the steric hindrance of the radical intermediates and thus retard undesired pinacol coupling. Based on this hypothesis, we started the investigation of reductive carboxylation with 4-acetylbiphenyl 1a as a model substrate (Fig. 3 ). When we used Cs 2 CO 3 as base, i Pr 2 NEt as the electron donor and N , N -dimethylformamide (DMF) as solvent (entry 1), the desired product 2a was obtained in 36% yield along with pinacol 2a ′ in 54% yield. We were pleased to find that the use of triethylsilylchloride (TESCl) as an additive significantly improved the selectivity to afford 2a in 52% yield and 2a ′ in 29% yield (entry 2). After systematic screening of different bases, solvents, chlorosilanes, and other Lewis acids (entries 3–9. Please see Supplementary Information ( SI) for more details), we found that the combination of trimethylsilylchloride (TMSCl) as additive, KO t Bu as base, and N , N -dimethylacetamide (DMA) as solvent was the best choice to give 2a in 80% isolated yield (entry 7). Control experiments indicated that all of the components (PC, base, TMSCl, i Pr 2 NEt, light, and CO 2 ) played crucial roles in this successful transformation (entries 10–15). Fig. 3: Reaction optimization. a Reaction conditions: 1a (0.2 mmol), Ir(ppy) 2 (dtbbpy)PF 6 (1.0 mol %), base (2.0 equiv), i Pr 2 NEt (2.0 equiv), additive (1.0 equiv) in solvent (2.0 mL) at room temperature (RT) in CO 2 atmosphere under irradiation with 30 W blue LED for 12 h. The corresponding reductive product alcohol, 1-([1,1′-biphenyl]-4-yl)ethan-1-ol 2a ″, was observed as a minor byproduct in generally lower than 10% yield. b Yields were determined by UPLC analysis with 1,1′-biphenyl as internal standard. The isolated yields are given in parentheses. c Chlorosilane (1.3 equiv). d Without light. e Without Ir(ppy) 2 (dtbbpy)PF 6 . f Without i Pr 2 NEt. g Under N 2 atmosphere. n.d. not detected, LED light-emitting diode, DMSO dimethyl sulfoxide, dtbbpy 4,4′-di- tert -butyl-2,2′-bipyridine, ppy 2-phenylpyridine, TMS trimethylsilyl. Full size image With appropriate reaction conditions in hand, we began to explore the substrate scope of alkyl aryl ketones, which are prone to undergo α-carboxylation [63] and homo-aldol reaction [64] in the presence of base. To our delight, as shown in Fig. 4 , ketones bearing different alkyl groups, such as methyl ( 1a , 1f , 1g , 1h , 1k , 1l ), ethyl ( 1b ), n -butyl ( 1c ), isopropyl ( 1d ), tert -butyl ( 1e ), cyclohexyl ( 1i ), and benzyl ( 1j ), all underwent the umpolung carboxylation selectively. Although increased steric hindrance on the alkyl groups induced lower reactivity, the desired products ( 2d , 2e , 2i ) were obtained in good yields when 2,4,6-tris(diphenylamino)-3,5-difluorobenzonitrile (3DPA2FBN) was used as the photocatalyst. Notably, the umpolung carboxylation of the challenging substrate 1i with CO 2 to give 2i , which is a key motif in oxybutynin (Fig. 2 ), had not been realized previously [21] . In addition to substrate 1h , which is activated with an electron-withdrawing group (EWG), the effective conversion of substrates 1k and 1l bearing higher reduction potential (e.g., 1k ( E 1/2 red = −2.1 V vs SCE)) could be achieved by using stronger reductive photosensitizer (3DPA2FBN, E 1/2 red = −1.92 V vs SCE) [66] , especially in the presence of TMSCl as carbonyl activating reagent. Moreover, esters ( 1h ), methoxy groups ( 1l ), naphthalene ( 1f ), and thiophene ( 1g ) moieties were tolerated under the reaction conditions. However, the dialkyl ketones and aldehydes, such as 4-phenylbutan-2-one and 3-phenylpropanal, were performed in standard condition, no desirable products were detected so far. It is presumably due to the higher reduction potential of the dialkyl ketones and alkyl aldehydes. Fig. 4: Substrate scope of alkyl aryl ketones. The standard conditions were used, as shown in Fig. 3 , entry 7. Isolated yields of corresponding carboxylic acids 2 are shown. a Using 3DPA2FBN (2.0 mol %) instead of Ir(ppy) 2 (dtbbpy)PF 6 . b KO t Bu (2.5 equiv), DMA (4 mL). Full size image Considering the importance of α-hydroxycarboxylic acids bearing two aryl groups, we further applied our catalytic system to the carboxylation of diaryl ketones (Fig. 5 ). Due to the higher reactivity and fewer side reactions, these substrates could undergo reductive carboxylation smoothly under milder reaction conditions. A variety of functional groups, such as trifluoromethyl ( 3e ), fluoro ( 3f , 3l , 3o ), chloro ( 3g , 3m ), and methoxyl ( 3d ), were tolerated at the para position of non-symmetric or symmetric diaryl ketones. Moreover, benzophenones bearing meta - ( 3h , 3i ) or ortho -substitutions ( 3j , 3k ) could afford the corresponding products in moderate to high yields (56–90%). Notably, the carboxylation of the benzylic C–H bond in 3k was not observed through HAT process by ketyl radical [67] . In addition to benzophenones, this method could be expanded to xanthone 3p , 2-benzoylthiophene 3q and di(thiophen-2-yl)methanone 3r . Fig. 5: Substrate scope of diaryl ketones. Reaction condition: ketones (0.2 mmol), Ir-catalyst (0.001 mmol), Cs 2 CO 3 (0.4 mmol), i Pr 2 NEt (0.3 mmol), DMF (2 mL), isolated yields of corresponding carboxylic acids, or methyl esters 4 are shown. a i Pr 2 NEt (1.0 equiv). Full size image As α-hydroxymalonic acid (tartronic acid) derivatives are important motifs in a range of natural products, the development of methods to synthesize them is imperative. The construction of such motifs via the umpolung carboxylation of α-ketoesters with CO 2 has not been reported. Therefore, we further tried to apply this strategy in generation of α-hydroxymalonic acid derivatives. To our delight, this catalytic system worked well for selective umpolung carboxylation of α-ketoesters (Fig. 6 ). The challenging sterically hindered tert -butyl-substituted α-ketoester 5a showed good reactivity under standard reaction conditions to give the desired product 6a in 75% yield. Moreover, α-ketoesters bearing secondary ( 5b ) and primary alkyl groups ( 5c – 5e ) also were suitable substrates to afford the desired products in moderate to good yields. Notably, an α-hydroxymalonic acid derivative containing a cholesterol moiety ( 6f ) was selectively obtained albeit in a diminished yield, demonstrating potential application of this strategy for late-stage diversification under mild conditions. Fig. 6: Substrate scope of α-ketoesters and α-ketoamides. 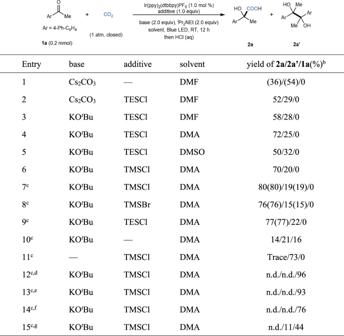Fig. 3: Reaction optimization. aReaction conditions:1a(0.2 mmol), Ir(ppy)2(dtbbpy)PF6(1.0 mol %), base (2.0 equiv),iPr2NEt (2.0 equiv), additive (1.0 equiv) in solvent (2.0 mL) at room temperature (RT) in CO2atmosphere under irradiation with 30 W blue LED for 12 h. The corresponding reductive product alcohol, 1-([1,1′-biphenyl]-4-yl)ethan-1-ol2a″, was observed as a minor byproduct in generally lower than 10% yield.bYields were determined by UPLC analysis with 1,1′-biphenyl as internal standard. The isolated yields are given in parentheses.cChlorosilane (1.3 equiv).dWithout light.eWithout Ir(ppy)2(dtbbpy)PF6.fWithoutiPr2NEt.gUnder N2atmosphere. n.d. not detected, LED light-emitting diode, DMSO dimethyl sulfoxide, dtbbpy 4,4′-di-tert-butyl-2,2′-bipyridine, ppy 2-phenylpyridine, TMS trimethylsilyl. The standard conditions were used, as shown in Fig. 3 , entry 7. Isolated yields of corresponding carboxylic acids or methyl esters 6 are shown. a Isolated yield of corresponding benzoate ester upon work up with BzCl. Bz benzoyl. Full size image Based on the success of α-ketoesters, we further tested the umpolung carboxylation of α-ketoamides with CO 2 , a process which has never been reported. Indeed, N -alkyl- N -aryl amides ( 5g – 5j ) and N , N -dialkyl amide ( 5k ) also reacted under the standard reaction conditions to afford the corresponding α-hydroxyamides in moderate yields. The steric hindrance of the alkyl group did not significantly affect the reaction, as demonstrated by the comparable yields for the carboxylations of N -alkyl- N -aryl amides ( 5g – 5j ). However, amides containing an N – H bond were not suitable substrates at this stage, which might because of the increased electron density of the carbonyl and/or the competitive quenching of deprotonated form of secondary amide with respect to i Pr 2 NEt. After demonstrating the viability of different kinds of ketones, we turned our attention to more challenging aryl aldehydes. Although umpolung carboxylations of aryl aldehydes with CO 2 are rare [43] , [68] , [69] , α-hydroxycarboxylic acids synthesis typically suffer from low yields, low selectivity, and limited scope. When aryl aldehydes were applied as substrates to the standard reaction conditions, we observed a complicated mixture of products due to intense side reactions, including pinacol coupling and disproportionation, which might arise from the lower steric hindrance of aldehydes and the strong base. In order to prevent such side reactions, we further tested several bulky chlorosilanes and weak bases. After systematic screening, we were pleased to find a suitable option using potassium pivalate (KOPiv) as base and Ph 3 SiCl as additive (Fig. 7 ). Under these modified reaction conditions, umpolung carboxylation of 7a took place smoothly to afford, after esterification, the desired product 8a in 60% yield along with 33% of pinacol 8a ′ . In contrast, 8a could only be obtained in 8% yield along with 63% of 8a ′ in the absence of Ph 3 SiCl, which indicates the significance of Ph 3 SiCl to the carboxylation of aryl aldehydes. Several aryl aldehydes bearing different substituents, including thiol ether ( 7c ) and thiophene ( 7d ), reacted to give the desired α-hydroxycarboxylic esters in 30 min with moderate to good yields. Moreover, fused aryl aldehydes, such as 2-naphthaldehyde ( 7e ) and phenanthrene-9-carboxaldehyde ( 7f ), also reacted well. Fig. 7: Substrate scope of aryl aldehydes. Isolated yields of corresponding methyl esters are shown. Full size image To gain more mechanistic insight into this transformation, we conducted several control experiments. As silyl enol ether 1A can be prepared easily from ketone 1a and TMSCl in the presence of base, we wondered whether it might act as the reaction intermediate. However, we failed to detect 1A at different stages of the standard reaction of 1a . To further confirm the assumption, we synthesized 1A and then applied it as the starting material for the carboxylation in the absence of TMSCl (Fig. 8a ). We found that a lower yield of the desired product 2a-Me was generated along with the dimethyl 2-hydroxy-2-phenylsuccinate 9 , which was never detected in the standard reaction of 1a , as a major byproduct. We hypothesized that the formation of 9 might involve the successive single electron transfer (SSET) reduction and carboxylation processes of the silyl enol ether 1A with CO 2 [70] . Moreover, we observed the full decomposition of 1A under a N 2 atmosphere to give 1a in 53% yield, indicating that the formation of 2a from 1A and CO 2 might proceed with 1a as the real reactant. Meanwhile, we observed that the reduction potential of 1A was slightly higher than 1a (see below). Therefore, we excluded the possibility that silyl enol ether 1A is the key intermediate in the observed umpolung carboxylation. Moreover, alcohol 2a ″ and TMS-protected 2a ″ were treated with standard conditions, 2a was not observed, 2a ″ and some dehydroxylative byproducts were detected, which rule out the direct C–H carboxylation pathway (please see the SI for details). Fig. 8: Control experiments. Isolated yields are shown. a Investigation of the possibility with sily enol ether 1A as intermediate. b Investigation of the effect of radical scavenger in the reaction. c Investigation of the effect of D 2 O in the reaction. a KO t Bu (1.0 equiv) was used. Full size image To further explore other intermediates in the reaction, we added a radical scavenger, 2,2,6,6-tetramethylpiperidinooxy (TEMPO), to the reaction of 1a under the standard conditions (Fig. 8b ). In the presence of TEMPO, the reaction was completely suppressed, indicating that radicals might be involved in this reaction. Furthermore, we tested the effect of D 2 O on the carboxylation reaction. The generation of 2a ″ from 1a was inhibited by the addition of D 2 O, thus precluding the determination of deuterium incorporation (please see the SI for details). The reaction of 3b in the presence of different amounts of D 2 O as additive, however, did provide alcohol 4b ″ in up to 83% yield and 70% deuterium incorporation (Fig. 8c ), suggesting that the benzylic carbanion is a possible intermediate. To demonstrate that the activation of carbonyl groups by a Lewis acidic chlorosilane is a critical part of the reaction, we performed Stern–Volmer luminescence studies and electrochemistry investigations (please see the SI for details). The luminescence of Ir(ppy) 2 (dtbbpy)PF 6 at λ max = 570 nm was readily quenched by i Pr 2 NEt with a slope of 266.4 (Fig. 9a ), which is much more significant than ketone 1a (−2.3) and TMSCl (51.2). These results suggest that the reaction proceeds with reductive quenching to give reduced Ir II -catalyst ( E 1/2 Red [Ir III /Ir II ] = −1.51 V vs SCE) [71] . Moreover, the cyclic voltammetry (CV) test (Fig. 9b ) indicated that the presence of TMSCl promoted reduction of the carbonyl by lowering the reductive potential. Thus, we believe that the SET reduction of the TMSCl-activated ketone 1a is favored to give the corresponding α-silyloxyl benzyl radical [72] , [73] , which might be further reduced by the Ir II -catalyst to generate a benzylic carbon anion. The following nucleophilic attack to CO 2 would give the corresponding products (Fig. 9c ). Fig. 9: Mechanistic experiments and proposed mechanism. a Stern-Volmer experiment. 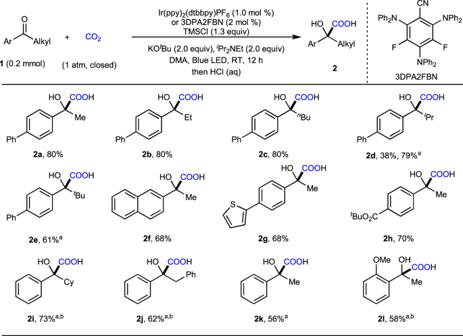Fig. 4: Substrate scope of alkyl aryl ketones. The standard conditions were used, as shown in Fig.3, entry 7. Isolated yields of corresponding carboxylic acids2are shown.aUsing 3DPA2FBN (2.0 mol %) instead of Ir(ppy)2(dtbbpy)PF6.bKOtBu (2.5 equiv), DMA (4 mL). b Cyclic voltammetry (CV) tests. c Proposed mechanism. Full size image In order to test other alternative pathways, such as coupling between benzyl radicals and a CO 2 radical anion, we further detected the formation of formate from CO 2 . Although a turnover number (TON) of 43 for the generation of formate was observed in the absence of ketones, the reduction of CO 2 was significantly depressed under the standard reaction of 1a (please see the SI for details). Meanwhile, the standard reduction potential of CO 2 in dry DMF is −2.21 V vs SCE [74] . The reduction potentials of 1a , 1k , and 7a in DMF are −1.81 V vs SCE, −2.1 V vs SCE, and −1.76 V vs SCE (please see the SI for details). Moreover, the reduction potential of α-ketoesters (for methyl 3-methyl-2-oxobutanoate, E 1/2 red = −1.75 V vs SCE [75] ) is also lower than CO 2 . These results indicated that the selective reduction of ketones over CO 2 . With this methodology in hand, we further demonstrated its utility by testing the gram-scale reaction and the synthesis of valuable intermediates and bioactive compounds (Fig. 10 ). First of all, we were delighted to find that the gram-scale reaction of 3a (6.0 mmol) proceeded well with comparable yield and efficiency (Fig. 10a ). Second, the product 2i could be reduced by LiAlH 4 to give diol 10 , which underwent cyclization to generate 1,3-dioxolane-2-thione 11 in a good yield (Fig. 10b ) [76] . The esterification of 2i and the following fluorination of the C–O bond generated α-fluorocarboxylic ester 12 [77] . Importantly, 2i could be transformed easily to bioactive oxypheonium 14 . In addition, the cyclization of 8a with isocyanate could give oxazolidine-2,4-dione 15 [78] . Moreover, as shown in Fig. 1 , the product 4a could be readily converted into valuable anticholinergic drugs trospium chloride (Sanctura) [24] , [27] , mepenzolate bromide (Cantil) [23] , and benactyzine [29] . The α-hydroxycarboxylic acid 4r is also a synthetic precursor for the drugs tiotropium bromide (Spiriva) and aclidinium bromide (Tudorza) [28] . 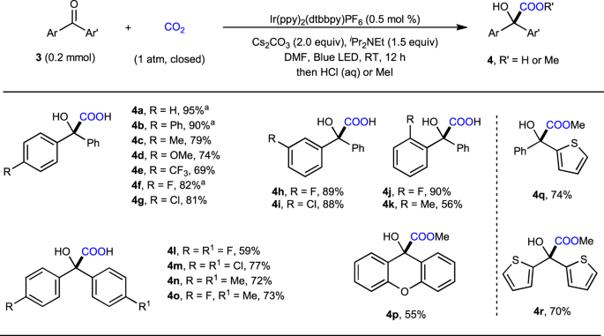Fig. 5: Substrate scope of diaryl ketones. Reaction condition: ketones (0.2 mmol), Ir-catalyst (0.001 mmol), Cs2CO3(0.4 mmol),iPr2NEt (0.3 mmol), DMF (2 mL), isolated yields of corresponding carboxylic acids, or methyl esters4are shown.aiPr2NEt (1.0 equiv). Fig. 10: Synthetic applications. a Gram-scale reaction. b Diverse functionalizations of products. (a) LiAlH 4 , THF, reflux. (b) TCDI, DCM, RT. (c) TMSCHN 2 , MeOH/Et 2 O; (d) Deoxofluor, DCM, RT, N 2 . (e) diethylamine, Na 2 CO 3 , DCE. (f) MeI, CH 3 CN, 65 °C. (g) p -Me-C 6 H 4 NCO, DMAP, THF, RT − 50 °C. TCDI = 1,1′-Thiocarbonyldiimidazole. 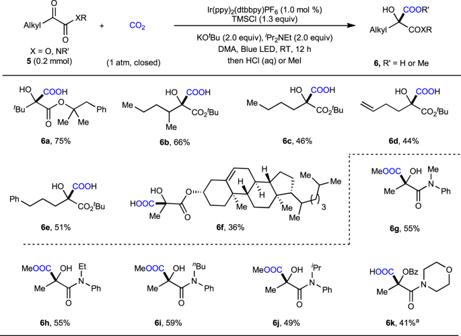Fig. 6: Substrate scope of α-ketoesters and α-ketoamides. The standard conditions were used, as shown in Fig.3, entry 7. Isolated yields of corresponding carboxylic acids or methyl esters6are shown.aIsolated yield of corresponding benzoate ester upon work up with BzCl. Bz benzoyl. DCM dichloromethane, Deoxofluor Bis(2-methoxyethyl)aminosulfur trifluoride, DMAP N , N -dimethylpyridin-4-amine, THF tetrahydrofuran. Full size image In this work, we developed a strategy for the visible-light photoredox-catalyzed umpolung carboxylation of carbonyl groups with CO 2 by using Lewis acidic chlorosilanes as activating/protecting groups. This strategy is general and practical for the carboxylation of diverse carbonyl compounds, including alkyl aryl ketones, diaryl ketones, α-ketoamides, α-ketoesters, and aryl aldehydes, to give valuable α-hydroxycarboxylic acids. The utility of this method is highlighted by facile generation of key intermediates to produce many drugs and natural products, including oxypheonium, mepenzolate bromide, benactyzine, and tiotropium. Moreover, this transformation features low catalyst loading, high selectivity, broad substrate scope, good functional group tolerance, mild reaction conditions (room temperature, 1 atm), and facile gram-scale reaction. The control experiments demonstrated the important role of chlorosilanes to promote the reaction and excluded the possibility of silyl enol ethers serving as key intermediates. Finally, carbon radicals and carbanions might be involved in this transformation. Synthesis of 2a – 2l and 6a – 6k The oven-dried Schlenk tube (10 mL) containing a stirring bar was charged with ketone (0.2 mmol), Ir(ppy) 2 (dtbbpy)PF 6 (1.9 mg, 1 mol %), or 3DPA2FBN (2.6 mg, 0.004 mmol), then added t BuOK (44.9 or 60.9 mg, 0.4 or 0.5 mmol) in glovebox. The tube was taken out, evacuated, and back-filled with CO 2 for three times. Subsequently, i Pr 2 NEt (66 μL, 0.4 mmol), TMSCl (34 μL, 0.26 mmol), and DMA (2 or 4 mL) were added via syringe under CO 2 atmosphere. Once added, the Schlenk tube was sealed at atmospheric pressure of CO 2 (1 atm). The reaction was stirred in water bath and irradiated with a 30 W blue LED lamp (3 cm away, with cooling fan to keep the reaction temperature at 25–30 °C) for 12 h. After completion, 0.5 mL n Bu 4 NF (1.0 N in THF) was carefully added to quench the reaction, the mixture was allowed to stir for 30 min at room temperature. Then, Work-up 1: the mixture was quenched with HCl (2 N), extracted with EtOAc, the combined organic phases were concentrated in vacuo. The residue was purified by silica gel flash chromatography (0.1% AcOH in petroleum ether/EtOAc) to give the corresponding α-hydroxycarboxylic acids as products. Or Work-up 2: MeI (37 μL, 3.0 equiv) was added via syringe. The resulting mixture was further stirred for 3 h at 60 °C. After cooling to room temperature, the mixture was quenched with HCl (2 N), extracted with EtOAc, the combined organic phases were concentrated in vacuo. The residue was purified by silica gel flash column chromatography (petroleum ether/EtOAc 100/1-50/1) to give the pure desired methyl α-hydroxycarboxylates. Synthesis of 4a – 4r The oven-dried Schlenk tube (10 mL) containing a stirring bar was charged with ketone (0.2 mmol), Ir(ppy) 2 (dtbbpy)PF 6 (1.0 mg, 0.001 mmol, 0.5 mol %), then added Cs 2 CO 3 (130.0 mg, 0.4 mmol) in glovebox. The tube was taken out, evacuated, and back-filled with CO 2 for three times. Subsequently, i Pr 2 NEt (33 or 50 μL, 0.2 or 0.3 mmol), DMF (2 mL) was added via syringe under CO 2 atmosphere. Once added, the Schlenk tube was sealed at atmospheric pressure of CO 2 (1 atm.). Then the work-up procedures were the same as above mentioned. Synthesis of 8a – 8f The oven-dried Schlenk tube (25 mL) containing a stirring bar was charged with aldehyde (0.2 mmol), Ir(ppy) 2 (dtbbpy)PF 6 (1.9 mg, 0.002 mmol, 1 mol %), Ph 3 SiCl (76.7 mg, 0.26 mmol), and PivOK (84.1 mg, 0.6 mmol) in glovebox. The tube was taken out, evacuated, and back-filled with CO 2 for three times. Subsequently, i Pr 2 NEt (66 μL, 0.4 mmol) and DMA (6 mL) were added via syringe under CO 2 atmosphere. Once added, the Schlenk tube was sealed at atmospheric pressure of CO 2 (1 atm.). After completion, 0.5 mL n Bu 4 NF (1.0 N in THF) was carefully added to quench the reaction, the mixture was quenched with HCl (2 N), extracted with EtOAc, the combined organic phases were concentrated in vacuo. 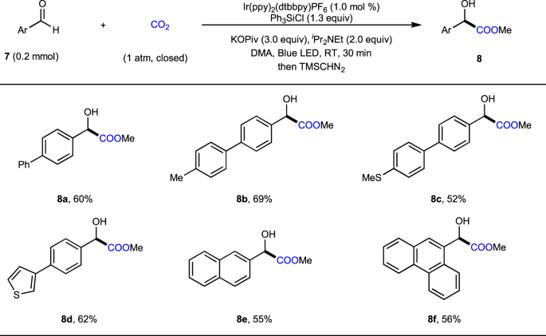Fig. 7: Substrate scope of aryl aldehydes. Isolated yields of corresponding methyl esters are shown. The crude residue was dissolved in 4 mL MeOH/Et 2 O (1/3), TMSCHN 2 (0.3 mL, 0.6 mmol, 2 M in hexanes) was added drop wisely at 0 °C. Upon completion. 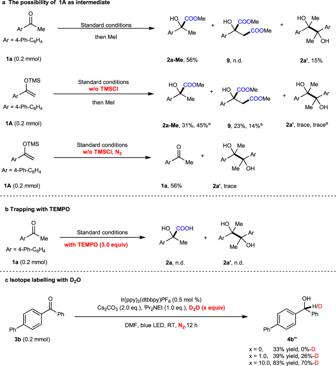Fig. 8: Control experiments. Isolated yields are shown.aInvestigation of the possibility with sily enol ether1Aas intermediate.bInvestigation of the effect of radical scavenger in the reaction.cInvestigation of the effect of D2O in the reaction.aKOtBu (1.0 equiv) was used. 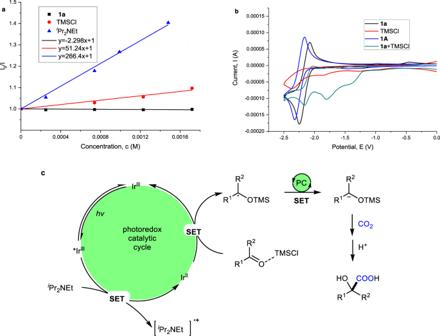Fig. 9: Mechanistic experiments and proposed mechanism. aStern-Volmer experiment.bCyclic voltammetry (CV) tests.cProposed mechanism. 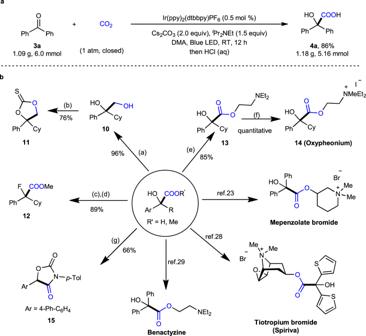Fig. 10: Synthetic applications. aGram-scale reaction.bDiverse functionalizations of products. (a) LiAlH4, THF, reflux. (b) TCDI, DCM, RT. (c) TMSCHN2, MeOH/Et2O; (d) Deoxofluor, DCM, RT, N2. (e) diethylamine, Na2CO3, DCE. (f) MeI, CH3CN, 65 °C. (g)p-Me-C6H4NCO, DMAP, THF, RT − 50 °C. TCDI = 1,1′-Thiocarbonyldiimidazole. DCM dichloromethane, Deoxofluor Bis(2-methoxyethyl)aminosulfur trifluoride, DMAPN,N-dimethylpyridin-4-amine, THF tetrahydrofuran. After removal of the solvent, the crude reaction mixture was purified on silica gel (petroleum ether and ethyl acetate) to afford the desired methyl α-hydroxycarboxylates.